Oxidation of difluorocarbene and subsequent trifluoromethoxylation As a versatile intermediate, difluorocarbene is an electron-deficient transient species, meaning that its oxidation would be challenging. Herein we show that the oxidation of difluorocarbene could occur smoothly to generate carbonyl fluoride. The oxidation process is confirmed by successful trifluoromethoxylation, 18 O-trifluoromethoxylation, the observation of AgOCF 3 species, and DFT calculations. Due to the unique properties of fluorine element such as strong electronegativity and small atomic radius, the incorporation of fluorine atom(s) into organic molecules could usually lead to profound changes of the latter’s physical, chemical, and biological properties [1] . Therefore, significant efforts have been directed towards the development of efficient methods for introducing fluorine or fluorinated moieties into organic compounds [2] , [3] . Difluorocarbene (:CF 2 ) has served as a versatile intermediate and the transformations of difluorocarbene has proved to be quite efficient for fluorine incorporation [4] , [5] . Typical difluorocarbene conversions, including insertions into X-H bonds (X=O, N, S, etc.) [4] , [6] , [7] , [2 + 1] cycloadditions with multi-bonds [8] , [9] , and coupling with other carbenes [10] , [11] , [12] , can conveniently construct various fluorinated functionalities, such as difluoromethyl, gem -difluorocyclopropyl and gem- difluoroalkenyl groups. However, these typical reactions are limited to the incorporation of a -CF 2 - moiety. We have previously found that difluorocarbene is so reactive that it can be readily trapped by a suitable sulfur [13] , [14] , [15] , selenium [16] , or nitrogen source [17] to generate thiocarbonyl fluoride (CF 2 =S), selenocarbonyl fluoride (CF 2 =Se), and cyanide anion (CN − ), respectively (Fig. 1a–c ). On the basis of these findings, which offers more possibilities for difluorocarbene chemistry, it is reasonable to conceive that the oxidation of difluorocarbene with a suitable oxygen source may proceed to afford carbonyl fluoride (CF 2 =O) (Fig. 1d ). Usually, oxidation reactions could proceed smoothly to oxidize electron-rich substrates, but not to electron-deficient substrates [18] , [19] . Since difluorocarbene is an electron-deficient transient intermediate [20] , its oxidation would be a challenging task. Furthermore, because CF 2 =O is a highly reactive gas and thus hard to detect, it cannot be determined simply by spectroscopic monitoring of the reaction whether the oxidation process occurs or not. Fig. 1 The transformations of difluorocarbene. a The transformation of difluorocarbene into thiocarbonyl fluoride. b The transformation of difluorocarbene into selenocarbonyl fluoride. c The transformation of difluorocarbene into cyanide anion. d The transformation of difluorocarbene into carbonyl fluoride. Full size image Herein we describe the oxidation of difluorocarbene by using diphenyl sulfoxide (Ph 2 S=O) as the oxidant to provide carbonyl fluoride, a process which is confirmed by successful trifluoromethoxylation and 18 O-trifluoromethoxylation reactions, the observation of AgOCF 3 species, and DFT calculations. A late-stage trifluoromethoxylation for the synthesis of a Trioxsalen derivative is shown to further demonstrate the synthetic utility of this trifluoromethoxylation protocol. 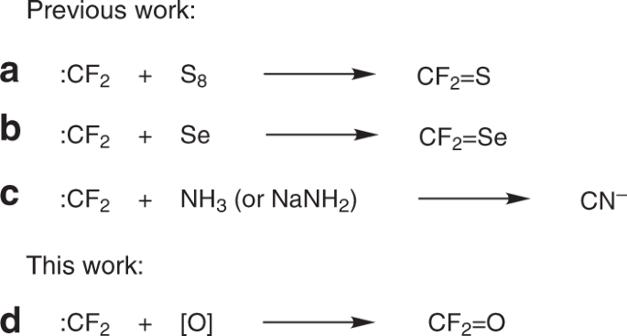Fig. 1 The transformations of difluorocarbene.aThe transformation of difluorocarbene into thiocarbonyl fluoride.bThe transformation of difluorocarbene into selenocarbonyl fluoride.cThe transformation of difluorocarbene into cyanide anion.dThe transformation of difluorocarbene into carbonyl fluoride. Optimization of the trifluoromethoxylation conditions Ph 3 P + CF 2 CO 2 − , developed by us recently [21] , and AgF were used as a difluorocarbene reagent and the fluoride source, respectively, in our efforts to ascertain the oxidation process via the trifluoromethoxylation of benzyl bromide 1-1 (Table 1 ). AgF was used to convert CF 2 =O into AgOCF 3 , which may be experimentally observed [22] to support the oxidation process. The oxidants were initially screened, but no desired trifluoromethoxylation product was detected in most cases (Table 1 , entries 1–5). To our delight, the use of DMSO (dimethyl sulfoxide) as the oxidant afforded the expected product in 9% yield (Table 1 , entry 6), suggesting that sulfoxides may be a suitable class of oxidants. We then examined other sulfoxides (Table 1 , entries 7–8) and diphenyl sulfoxide was found to be a superior choice (Table 1 , entry 8). Other fluoride sources, including inorganic (Table 1 , entries 9–11) and organic (Table 1 , entry 12, TBAF=tetra- n -butylammonium fluoride) fluoride salts, were examined, but they were all ineffective. This indicates that the Ag ion may play an important role in the reaction. A brief survey of reaction solvents (Table 1 , entries 13–17) showed that THF (tetrahydrofuran) or DCM (dichloromethane) was the suitable solvent for this conversion (Table 1 , entries 15 and 16). The use of 2,2′-bipyridine or a crown ether as a ligand (Table 1 , entries 18 and 19) significantly increased the product yield. A 67% yield was obtained if both bipyridine and the crown ether were present (Table 1 , entry 20). The concentration affected the reaction slightly, and the yield increased with increasing concentration (Table 1 , entry 21 vs entry 20). At this concentration, the yield decreased if either the crown ether or 2,2′-bipyridine was not used (Table 1 , entries 22−23). Table 1 Optimization of trifluoromethoxylation conditions. Full size table Mechanistic investigations Further experimental evidence was collected to support the difluorocarbene oxidation process. 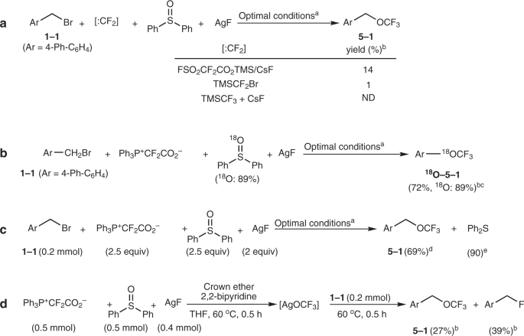Fig. 2 Mechanistic investigation.aThe use of other difluorocarbene reagents for trifluoromethoxylation.bThe identification of the oxygen source by18O-labeling.cThe identification of the oxygen source by isolating Ph2S.dThe confirmation of the AgOCF3complex.aThe optimal conditions are shown as Table1, entry 21: substrate1(0.2 mmol), Ph3P+CF2CO2−(2.5 equiv), Ph2S=O (2.5 equiv), AgF (2 equiv), 2,2′-bipyridine (1.5 equiv), and 2,3,11,12-dibenzo-18-crown-6 (0.5 equiv) in THF (1.5 mL) at 60 °C for 0.5 h;bYields were determined by19F NMR spectroscopy.cThe18O content was determined by EI-MS.dIsolated yield calculated based on substrate1–1.eIsolated yield based on Ph2S=O consumed. The use of other difluorocarbene reagents such as FSO 2 CF 2 CO 2 TMS [23] and TMSCF 2 Br [8] could also give the desired trifluoromethoxylation product, albeit in a low yield, suggesting that difluorocarbene is a key intermediate (Fig. 2a ). CF 2 =O could not be detected in the reaction mixtures, because it is a highly electrophilic species and would be rapidly attacked by AgF to provide AgOCF 3 . Even stirring the mixture of Ph 3 P + CF 2 CO 2 − and Ph 2 S=O alone could not lead to the observation of CF 2 =O, because CF 2 =O would easily react with the nucleophile, Ph 3 P generated from Ph 3 P + CF 2 CO 2 − [9] . Ph 2 S=O should be the oxygen source to oxidize difluorocarbene to generate CF 2 =O, since 18 O-labeled diphenyl sulfoxide afforded the CF 3 18 O product (Fig. 2b ), and diphenyl sulfoxide underwent deoxygenation to afford diphenyl sulfide (Ph 2 S) in a high yield based on Ph 2 S=O consumed (39% of Ph 2 S=O was recovered) (Fig. 2c ) ( Supplementary Methods ). A stepwise reaction was performed to confirm the generation of the AgOCF 3 complex (Fig. 2d ). Without the presence of a substrate, heating a mixture of Ph 3 P + CF 2 CO 2 − /Ph 2 S=O/AgF with ligands at 60 °C for 0.5 h led to the formation of a number of unkonwn species, as detected by 19 F NMR spectroscopy (Supplementary Fig. 2 ). Two broad signals, appearing at −21.66 and −21.94 ppm in the 19 F NMR spectrum, respectively, may correspond to two different ligand-coordinated AgOCF 3 complexes [22] . Subsequent addition of substrate 1–1 afforded the desired trifluoromethoxylation product, further supporting that AgOCF 3 was generated from the Ph 3 P + CF 2 CO 2 − /Ph 2 S=O/AgF system (Fig. 2d ). In addition to the trifluoromethoxylation product, a fluorination byproduct was observed (Fig. 2d ). However, almost no fluorination byproduct was observed under the optimal conditions (Table 1 , entry 21), which suggests that AgOCF 3 was too reactive and decomposed easily. Fig. 2 Mechanistic investigation. a The use of other difluorocarbene reagents for trifluoromethoxylation. b The identification of the oxygen source by 18 O-labeling. 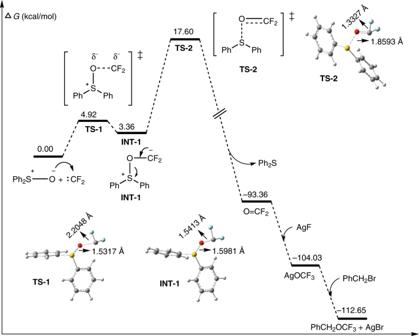Fig. 3 Relative free energies for difluorocarbene-oxidation-based trifluoromethoxylation. All calculations were performed in Gaussian 09 D01 package. c The identification of the oxygen source by isolating Ph 2 S. d The confirmation of the AgOCF 3 complex. a The optimal conditions are shown as Table 1 , entry 21: substrate 1 (0.2 mmol), Ph 3 P + CF 2 CO 2 − (2.5 equiv), Ph 2 S=O (2.5 equiv), AgF (2 equiv), 2,2′-bipyridine (1.5 equiv), and 2,3,11,12-dibenzo-18-crown-6 (0.5 equiv) in THF (1.5 mL) at 60 °C for 0.5 h; b Yields were determined by 19 F NMR spectroscopy. c The 18 O content was determined by EI-MS. d Isolated yield calculated based on substrate 1 – 1 . e Isolated yield based on Ph 2 S=O consumed. Full size image DFT calculations at the M062X//6–31 + + G(d,p)/LANL2DZ level provided insights into the mechanism of the oxidation of difluorocarbene and the subsequent trifluoromethoxylation. We have previously demonstrated that Ph 3 P + CF 2 CO 2 − is an efficient difluorocarbene precursor, and has proposed that difluorocarbene is generated via a decarboxylation process, i.e., Ph 3 P + CF 2 CO 2 − → Ph 3 P + CF 2 − → :CF 2 [14] , [15] , [24] . Calculations revealed that the activation energy for this process is quite low (10.12 kcal mol −1 ) (Supplementary Fig. 3 and Supplementary Data 1 ), supporting the mechanistic proposal. As an electron-deficient species, difluorocarbene can be attacked by Ph 2 S=O to form an O–CF 2 bond (Fig. 3 , INT-1 ). The formation of this bond weakens the S–O bond in Ph 2 S=O, as shown by the increasing S–O bond length from TS-1 to INT-1 . Back donation of the carbon lone pair strengthens the O–CF 2 bond and further weakens the S–O bond (Fig. 3 , TS-2 ). Complete cleavage of the S–O bond releases Ph 2 S and carbonyl fluoride (CF 2 =O), a process which is thermodynamically favored. CF 2 =O is electrophilic and is therefore trapped by AgF to generate AgOCF 3 , which can readily convert the substrates to the final products. The Ag ion can activate the substrates by precipitating the AgBr salt. Identification of transition state TS-2 enabled us to calculate the overall activation energy, i.e., 17.60 kcal mol −1 ; this value is low and in agreement with the rapid process. Fig. 3 Relative free energies for difluorocarbene-oxidation-based trifluoromethoxylation. All calculations were performed in Gaussian 09 D01 package. Full size image The introduction of CF 3 O installation The above results revealed that difluorocarbene could indeed be oxidized to give carbonyl fluoride. The oxidation of difluorocarbene and the subsequent trifluoromethoxylation provides an efficient protocol for CF 3 O incorporation. CF 3 O incorporation has received increasing attention because the CF 3 O group is a common structural motif in pharmaceuticals [25] , [26] , agrochemicals [27] , [28] , and functional materials [29] , [30] . A number of effective trifluoromethoxylation methods have been developed, including nucleophilic [31] , [32] , [33] , [34] , [35] , [36] , [37] , radical [38] , [39] , [40] , and transition-metal-promoted [41] , [42] , [43] , [44] reactions. As the use of a CF 3 O-containing reagent is required, these approaches cannot be directly applied to 18 O-labeling trifluoromethoxylation. Furthermore, the CF 3 O-containing reagents used are usually volatile, expensive, or difficult to prepare. In contrast, in the above protocol, CF 3 O moiety was formed from a reagent system consisting of Ph 3 P + CF 2 CO 2 − , which could be easily prepared and easy-to-handle, an oxygen source and fluoride anion. Apparently, this reaction provides a strategy for 18 O-labeling trifluoromethoxylation, which may be achieved by replacing the oxygen source with 18 O-source. 18 O-trifluoromethoxylation may show great value as 18 O-labeling has found widespread application in various research areas such as proteomics [45] , [46] , [47] and synthetic chemistry [48] , [49] , [50] . The substrate scope of trifluoromethoxylation Since difluorocarbene could be oxidized and the subsequent trifluoromethoxylation proceeded smoothly (Table 1 , entry 21), we then investigated the substrate scope of trifluoromethoxylation. 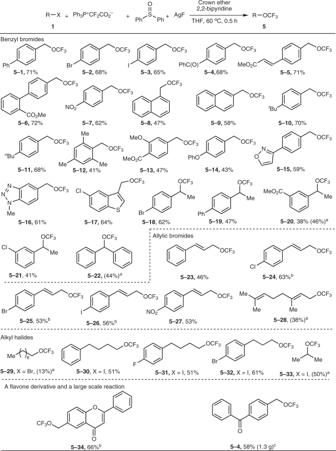Fig. 4 Difluorocarbene-oxidation-based trifluoromethoxylation. Isolated yields are shown. Reaction conditions: substrate1(0.8 mmol), Ph3P+CF2CO2−(2.5 equiv), Ph2S = O (2.5 equiv), AgF (2 equiv), 2,2′-bipyridine (1.5 equiv), and 2,3,11,12-dibenzo-18-crown-6 (0.5 equiv) in THF (6 mL) at 60 °C for 0.5 h.aThe yields in parentheses were determined by19F NMR spectroscopy.b0.2 mmol of substrate was used.c8 mmol of substrate was used. Figure 4 shows that electron-deficient, -neutral, and -rich benzyl bromides were all converted to the desired products in moderate to good yields ( 5–1 ~ 5–17 ). Various functional groups were tolerated, e.g., halide, ketone, ester, alkene, cyano, nitro, ether, and various heterocycles. Heterocycles usually have interesting physicochemical properties, and therefore the easy access to CF 3 O-containing heterocycles could be useful in the life sciences ( 5–15 ~ 5–17 ). Transformation of secondary benzyl bromides gave moderate yields ( 5–18 ~ 5–22 ). The diphenyl substituted product ( 5–22 ) was unstable, and a heterolytic cleavage of the C–OCF 3 bond readily occurred to form a diphenyl-stabilized methyl cation, hydrolysis of which led to an alcohol by product (Ph 2 CH-OH) in 35% isolated yield. In addition to benzyl bromides, allyl bromides were also converted under these conditions ( 5–23 ~ 5–28 ). The reactivity of alkyl bromide ( 5–29 ) was much lower than that of benzyl bromides. Alkyl iodides ( 5–30 ~ 5–33 ) underwent the desired reaction smoothly to give the expected products in moderate yields. A method for achieving direct access to a flavone derivative was developed ( 5–34 ) and a moderate yield was obtained for a large-scale reaction ( 5–4 ), demonstrating the synthetic utility of this trifluoromethoxylation protocol. Fig. 4 Difluorocarbene-oxidation-based trifluoromethoxylation. Isolated yields are shown. Reaction conditions: substrate 1 (0.8 mmol), Ph 3 P + CF 2 CO 2 − (2.5 equiv), Ph 2 S = O (2.5 equiv), AgF (2 equiv), 2,2′-bipyridine (1.5 equiv), and 2,3,11,12-dibenzo-18-crown-6 (0.5 equiv) in THF (6 mL) at 60 °C for 0.5 h. a The yields in parentheses were determined by 19 F NMR spectroscopy. b 0.2 mmol of substrate was used. c 8 mmol of substrate was used. Full size image Trioxsalen, a furanocoumarin and a psoralen derivative obtained from plants, can be used for phototherapy treatment of vitiligo and hand eczema [51] . A convenient route to the CF 3 O-containing Trioxsalen derivative ( 8 ) was developed to further show the synthetic utility of this trifluoromethoxylation strategy. The trifluoromethoxylation of the precursor ( 7 ), prepared from the commercially available m -benzenediol by a reported procedure (Supplementary Fig. 1 ) [52] , [53] , occurred smoothly to give the Trioxsalen derivative in a moderate yield (Fig. 5 ). Fig. 5 The synthesis of CF 3 O-containing Trioxsalen derivative. The derivative was synthesized by a late-stage trifluoromethoxylation reaction. Full size image 18 O-Trifluoromethoxylation 18 O-Labeling trifluoromethoxylation is challenging, because all reported trifluoromethoxylation methods have to use a CF 3 O-containing reagent and the corresponding CF 3 18 O-reagents are difficult to prepare. 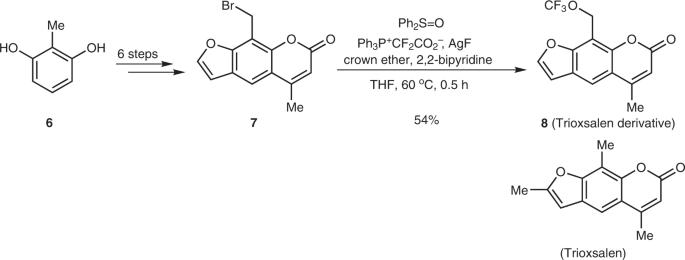Fig. 5 The synthesis of CF3O-containing Trioxsalen derivative. The derivative was synthesized by a late-stage trifluoromethoxylation reaction. 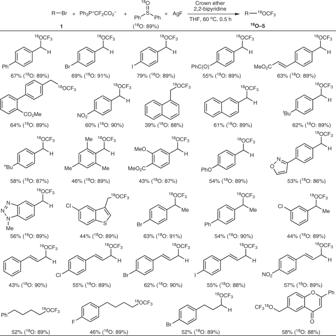Fig. 6 Difluorocarbene-oxidation-based18O-trifluoromethoxylation. Isolated yields. Reaction conditions: substrate1(0.2 mmol), Ph3P+CF2CO2−(2.5 equiv), Ph2S=18O (2.5 equiv), AgF (2 equiv), 2,2′-bipyridine (1.5 equiv), and 2,3,11,12-dibenzo-18-crown-6 (0.5 equiv) in THF (1.5 mL) at 60 °C for 0.5 h. The18O contents were determined by EI-MS. Recently, Tang used an 18 O-labeled reagent, ArSO 2 – 18 OCF 3 , to explore and elucidate the mechanism of the trifluoromethoxylation reaction; only a 33% 18 O content was obtained in the desired product [37] . They proposed that the low 18 O-content was because of the 16 O- 18 O exchange in the SO 2 – 18 OCF 3 moiety from the reagent. We employed 18 O-labeled diphenyl sulfoxide (Ph 2 S= 18 O, 18 O content: 89%) as the oxygen source in this difluorocarbene-oxidation-based trifluoromethoxylation reaction. Since the reagent, Ph 2 S= 18 O, did not contain any 16 O atom, no 16 O- 18 O exchange would occur and therefore the expected products were obtained with high 18 O contents (Fig. 6 ). Fig. 6 Difluorocarbene-oxidation-based 18 O-trifluoromethoxylation. Isolated yields. Reaction conditions: substrate 1 (0.2 mmol), Ph 3 P + CF 2 CO 2 − (2.5 equiv), Ph 2 S= 18 O (2.5 equiv), AgF (2 equiv), 2,2′-bipyridine (1.5 equiv), and 2,3,11,12-dibenzo-18-crown-6 (0.5 equiv) in THF (1.5 mL) at 60 °C for 0.5 h. The 18 O contents were determined by EI-MS. Full size image In summary, we have shown that difluorocarbene could be oxidized to afford carbonyl fluoride. This process was confirmed by the successful trifluoromethoxylation, 18 O-trifluoromethoxylation, the observation of AgOCF 3 species, and DFT calculations. It is worth noting that the 18 O-products were obtained with high 18 O-contents. A CF 3 O-containing Trioxsalen derivative was synthesized by this trifluoromethoxylation protocol. The oxidation of difluorocarbene may provide more possibilities for difluorocarbene chemistry. Typical procedure for trifluoromethoxylation Into a 20 mL sealed tube were added benzyl bromide 1–1 (0.8 mmol, 197.7 mg, 1.0 equiv), Ph 3 P + CF 2 CO 2 − (2.0 mmol, 712.0 mg, 2.5 equiv), Ph 2 S=O (2.0 mmol, 404.6 mg, 2.5 equiv), AgF (1.6 mmol, 203.2 mg, 2.0 equiv), 2,2′-bipyridine (1.2 mmol, 187.4 mg, 1.5 equiv), 2,3,11,12-dibenzo-18-crown-6 (0.4 mmol, 144.2 mg, 0.5 equiv), and THF (6 mL) under a N 2 atmosphere. The tube was sealed and the reaction mixture was stirred at 60 °C for 30 min. After the mixture was cooled to room temperature, the pure product was isolated by flash column chromatography. Typical procedure for 18 O-trifluoromethoxylation Into a 10-mL sealed tube were added benzyl bromide 1–1 (0.2 mmol, 49.4 mg, 1.0 equiv. ), Ph 3 P + CF 2 CO 2 − (0.5 mmol, 178.0 mg, 2.5 equiv), Ph 2 S= 18 O (0.5 mmol, 102.1 mg, 2.5 equiv), AgF (0.4 mmol, 51.0 mg, 2.0 equiv), 2,2′-bipyridine (0.3 mmol, 47.0 mg, 1.5 equiv), 2,3,11,12-dibenzo-18-crown-6 (0.1 mmol, 36.0 mg, 0.5 equiv), and THF (1.5 mL) under a N 2 atmosphere. The tube was sealed and the reaction mixture was stirred at 60 o C for 30 min, and the mixture was cooled to room temperature. The pure product was isolated by flash column chromatography, and the 18 O contents were determined by GC-MS (EI) spectroscopy. For the preparation of starting materials and the characterization data of the products, see Supplementary Methods . For the NMR spectra of the compounds, see Supplementary Figs. 5 – 184 . For EI spectra of the 18 O-products, see Supplementary Figs. 185 – 214 . For DFT calculations, see Supplementary Figs. 3 and 4 and Supplementary Data 1 and 2 .